Food web expansion and contraction in response to changing environmental conditions Macroscopic ecosystem properties, such as major material pathways and community biomass structure, underlie the ecosystem services on which humans rely. While ecologists have long sought to identify the determinants of the trophic height of food webs (food chain length), it is somewhat surprising how little research effort is invested in understanding changes among other food web properties across environmental conditions. Here we theoretically and empirically show how a suite of fundamental macroscopic food web structures respond, in concert, to changes in habitat accessibility using post-glacial lakes as model ecosystems. We argue that as resource accessibility increases in coupled food webs, food chain length contracts (that is, reduced predator trophic position), habitat coupling expands (that is, increasingly coupled macrohabitats) and biomass pyramid structure becomes more top heavy. Our results further support an emerging theoretical view of flexible food webs that provides a foundation for generally understanding ecosystem responses to changing environmental conditions. Food webs provide the architecture that underlies species diversity patterns, and thus mediate system dynamics [1] , [2] and determine key ecosystem functions (for example, nutrient cycling [3] and contaminant bioaccumulation [4] ). Often, in order to simplify these diverse systems, studies focus on dominant food chains [5] , [6] , [7] , and therefore food chain length is a common and successful metric for capturing ecosystem structure [8] , [9] . Nonetheless, recent work considers that food webs are not so isolated [10] , [11] , [12] , [13] and often higher-order mobile consumers couple food webs (that is, link food chains) in space [14] , [15] , [16] , [17] , [18] . The extent that mobile predators couple spatially distinct macrohabitats is a measure of spatial coupling width on the landscape. As such, habitat coupling can be thought of as a spatial analogue to food chain length. We consider habitat coupling to be maximal when distinct resource chains, in different habitats, are equally coupled. This approach combines both topology, increases in the number of links to new resource pathways, and interaction strength. According to this usage, in the absence of habitat coupling, a food web is a chain. Habitat coupling increases topologically by the linking of additional habitat resource chains and reaches a maximum width for a given topology when all distinct habitats are equally coupled. The extent that conditions mediate predator coupling across subsystems has potential implications for the general structure, function and persistence of ecosystems [14] , [19] . A recent response to the challenge of predicting ecosystem change considers how fundamental food web structures vary across conditions. Ecologists have long noticed that food chain lengths vary among ecosystems [6] and have sought to understand the primary determinants of these changes [7] , [20] , [21] , [22] , [23] , [24] , [25] . Empirical studies consistently find that at a regional level food chain length shortens with reduced ecosystem size [7] , [19] , [20] , [22] , [25] , [26] , yet the mechanisms for this relationship remain largely uncertain [9] . Diversity may have a role in this empirical outcome, as larger systems can be more diverse, and thus more likely to contain higher-order consumer species and longer food chains [7] . However, research also suggests that organism behaviour may functionally modify food chain length through changes in the amount of omnivory [9] , [19] , [22] . Omnivory may increase, for example, if a predator suppresses intermediate consumer densities through strong consumption, releasing shared prey to thrive. Now more numerous, these low trophic-position prey organisms are consumed in greater proportion thereby reducing predator trophic positions [19] . In addition to omnivory, habitat coupling strength can functionally alter food webs as coupling regulates the energy available to upper trophic levels (that is, predators) through access to novel production across habitats [14] , [15] , [19] . Given that space has a role in accessibility, changing spatial conditions may alter coupling and thus space can be an important regulator of production to upper trophic levels with implications for fundamental food web properties, such as dominant food chain length, omnivory and biomass structure. In what follows, we provide a process-driven theory for changes to a suite of key food web properties across different environmental conditions. Using a coupled food web approach, we develop a simple spatially implicit resource accessibility argument that extends core ecological concepts from food chains, trophic cascades and spatial food webs [5] , [9] , [12] . Notably, rather than a strict topological approach where feeding links are either present or absent, our theory generates empirically tractable top predator interaction strengths and trophic control. We then empirically test our theory with real food web data across two natural gradients that alter the spatial characteristics and thus the accessibility of lake systems: overall lake size and the relative size of the littoral habitat. Our approach is synthetic in that we draw from a number of published studies adding new data and analyses to develop our theory. To conclude, we discuss the general implications of changing food webs for ecosystem structure and sustainability in a rapidly changing world. Biological assumptions and the food web model Our general conjecture is that constraints (for example, physiological and morphological) often mediate prey susceptibility to predators, and that this susceptibility then varies across environmental conditions fundamentally altering an ecosystem's response to change. Recent research argues that food chain length and the coupling of habitats by mobile predators are influenced by ecosystem size [19] , [20] , [22] . Here, we present prey accessibility as a trait-mediated mechanism link to these phenomena to each other and to ecosystem biomass structure. From behavioural ecology, it is generally accepted that consumers cannot access the full population density of their prey under all conditions [27] . This is premised by the idea that predators are constrained to consume prey within their sensory capabilities (for example, their foraging scale) and the distribution of their prey. As such, prey may take refuge, elevating their densities, in areas that are difficult for predators to access. When facing restrictive conditions, predators may search less of the existing habitat and, therefore, prey find themselves in a refuge from predation in unsearchable habitat ( Fig. 1c ; Supplementary Fig. S1 ). This idea extends to a system-level context under the premise that larger ecosystems tend to have greater habitat heterogeneity [28] and thus more potential prey refugia compared with smaller ecosystems. Therefore, limited access across subhabitats may reduce prey availability in larger systems compared with those systems that are smaller. Based on these ideas, we further develop a general theory using an empirical case to help communicate model mechanics and our assumptions. 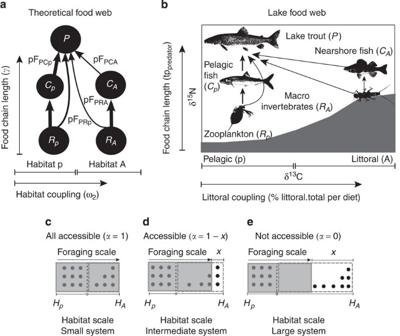Figure 1: Predicting food web structure from theory to nature. (a) Theoretical food web. Food chain length and spatial coupling depend on the direction (arrow) and relative proportion (thickness) of material flow,pF's, through feeding links calculated from equation (1).P,CandRdensities are represented by black circle size. Hatched lines delineate habitat boundaries. Hatched arrows on the axes show the direction of increasing food chain length and coupling strength. Symbols,γandω2, refer to food chain length and coupling strength estimates calculated using equations (6) and (9), respectively. (b) Lake food web structure. Pelagic and littoral resources chains, each containing fish and invertebrate prey, are coupled by lake trout. Chain dependence is delineated by stable isotope δ13C and vertical position in the web by δ15N (also calculated with stomach content data). Littoral coupling strength estimates are based on theCAandRAcontribution toP's total consumption. Food chain length is reported as predator trophic position (tppredator) (that is, trophic transfer between baseline production and predator of the sink web). (c–e) A conceptual model of accessibility. (c) Foraging scale (arrow) is equal to habitat scale (hatched lines), and all prey (black dots) are potentially accessible (shaded area). (d) At intermediate scales, a fraction of prey (x) is not accessible. Here, the highest prey density is located beyond the foraging scale of the predator. For completeness, we show the end point whereHAprey are not accessible to the predator (e). Dotted line visually separates habitats (HpandHA). Dashed box visually containsHAprey and if not shaded is not accessible. Figure 1: Predicting food web structure from theory to nature. ( a ) Theoretical food web. Food chain length and spatial coupling depend on the direction (arrow) and relative proportion (thickness) of material flow, pF 's, through feeding links calculated from equation (1). P , C and R densities are represented by black circle size. Hatched lines delineate habitat boundaries. Hatched arrows on the axes show the direction of increasing food chain length and coupling strength. Symbols, γ and ω 2 , refer to food chain length and coupling strength estimates calculated using equations (6) and (9), respectively. ( b ) Lake food web structure. Pelagic and littoral resources chains, each containing fish and invertebrate prey, are coupled by lake trout. Chain dependence is delineated by stable isotope δ 13 C and vertical position in the web by δ 15 N (also calculated with stomach content data). Littoral coupling strength estimates are based on the C A and R A contribution to P 's total consumption. Food chain length is reported as predator trophic position (tp predator ) (that is, trophic transfer between baseline production and predator of the sink web). ( c–e ) A conceptual model of accessibility. ( c ) Foraging scale (arrow) is equal to habitat scale (hatched lines), and all prey (black dots) are potentially accessible (shaded area). ( d ) At intermediate scales, a fraction of prey ( x ) is not accessible. Here, the highest prey density is located beyond the foraging scale of the predator. For completeness, we show the end point where H A prey are not accessible to the predator ( e ). Dotted line visually separates habitats ( H p and H A ). Dashed box visually contains H A prey and if not shaded is not accessible. Full size image The predatory fish, lake trout ( Salvelinus namaycush ), is an excellent example of an organism that exhibits this type of trait-mediated response to changing environmental conditions. Lake trout tend to reside in the cold pelagic zone of northern post-glacial lakes, avoiding the warm near-shore littoral habitat during the summer months. While lake trout forage on the cold-water pelagic food chain, they are still capable of making short foraging bouts into the warmer near-shore food chain [29] . Littoral coupling strength, however, depends on environmental conditions (for example, littoral habitat size) [30] . Small littoral habitats are readily accessible by lake trout even over a short foraging bout, while larger littoral habitats have areas that are thermally inaccessible. We derived a simple spatially implicit food web model based on three empirically motivated assumptions. Lake trout prefer cold-water habitats (8–12 °C) [31] , [32] , and so are thermally constrained to limited foraging bouts in the warm near-shore habitat during summer months ( ∼ 20 °C average summer water temperature at the southern end of their zoogeographic range) (A.1, Supplementary Discussion ). In the southern end of their distribution where most data are collected, for example, lake trout are capable of short foraging bouts into the warm littoral zone [29] . As prey distributions in the near-shore zone also tend to show the highest densities at the lake edge (A.2, Supplementary Fig. S2 ), the furthest distance from the deep pelagic habitat preferred by lake trout, littoral prey can be difficult to access by lake trout. In addition, the peak near-shore littoral prey density does not change in a predictable way across lakes (A.3, Supplementary Fig. S2 ). Given these physiological constraints and the prey spatial distribution, we argue that as the littoral warm-water habitat gets smaller, lake trout should be able to more easily access littoral prey. Similarly, as littoral habitat increases in size, prey should find themselves in thermal refugia from predatory lake trout. The general application of the above assumptions allows us to derive a spatially implicit scaling parameter, α , that links foraging scale to mean resource density and habitat size ( Supplementary Figs S1–S3 ). A unitless parameter, α , reflects the ratio that scales mean prey density available to total mean prey per density for a habitat and is derived from a constant area foraged, f , divided by total habita area, H A , ( H A , area foraged ( f )+area inaccessible ( I ); H A ≥ f ) such that when I =0, all resources are accessible, α=1 , and when α=0 resources are inaccessible ( Fig. 1c ; see Supplementary Figs S1 and S2 for full derviation). With this scaling parameter, we employ the following Lotka–Volterra model, with logistic resource growth, and linear functional responses to represent a three trophic-level spatially coupled food web ( Fig. 1a ): where, r i is the maximum intrinsic rate of increase for each resource for the preferred, p , and the alternate, A , habitats, respectively, and, K i , is the carrying capacity of each resource (density). The attack rate of the consumer on the resources is defined as a Ci Ri . Similarly, a PRi is the attack rate of the predator on each resource and a PCi , the predators attack rate on each consumer. Finally, Mc i and M P are the mortality rates for C i and P , and e C,P is the rate that prey are converted to C 's or P (for units see Supplementary Table S1 ). As discussed above, this food web model consists of a mobile predator, P , that forages on two distinct food chains each containing a consumer, C , and a resource, R ( Fig. 1a ). Biologically, the model includes the ability for food web structure to change in two important ways. First, the predators ability to forage in the alternative habitat depends on that habitat's size. Thus, changing alternative habitat size affects coupling strength into both habitats (that is, degree of habitat coupling) ( Fig. 1c ). Second, dynamic changes in predator densities P ultimately influence the densities of R to C in both habitats, and so drives a change in the amount of omnivory ( Fig. 1a ). As an example, if C is suppressed by elevated P densities with increased resource accessibility, then R is released to fluorish and P naturally begins to consume more prey lower in the food web. Such a scenario decreases food chain length and increases omnivory. The general, three-level, two-channel trophic structure of the theoretical structure above maps to natural lake trout food web topologically (equation. (1); Fig. 1a,b ; Methods). With the model system described above, equation (1), we conduct a theoretical experiment that changes the mean prey density available in a two-habitat system by effectively reducing one habitat's size. As size is reduced by increasing α , the model system becomes effectively smaller (move from right to left on the x axis Fig. 2 ) and the predator perceives prey in the alternative habitat compartment as more accessible. In a sense, changing the food web accessibility here has a direct influence on the amount of secondary habitat prey that can be consumed by the predator. Thus, our theory predicts (1) that as a secondary habitat is more accessible, predators consume more prey from that habitat and thus coupling increases ( Fig. 2a ). This secondary habitat coupling increase allows the predator population to increase its intake compared with the single habitat and now suppresses primary consumer prey. Notice that with strong top–down suppression in small systems, secondary consumers are low in density relative to their prey (owing to the top heavy pyramid; Fig. 2b ). So increased coupling drives a second prediction (2) that the trophic pyramid of the system shifts from the more classic Eltonian pyramid [6] to a more top heavy pyramid ( Fig. 2b ) with increased predator to consumer densities ( Fig. 2b inset). The changing biomass pyramid releases R relative to C . Thus, for small systems, the top predator has a greater propensity to feed on lower trophic levels (that is, feeds more on R that is high relative to C ). The consumption of R maintains the predator with the suppression of C and the accompanying reduction in C A production. This effect is our third prediction (3) that omnivory increases in small or high accessibility ecosystems ( Fig. 2c ). As omnivory increases, the predator is supported proportionally by more prey from lower trophic levels. From this result, we arrive at a fourth and final related prediction (4) that food web length contracts with decreases in ecosystem size (that is, increased omnivory; Fig. 2d ). 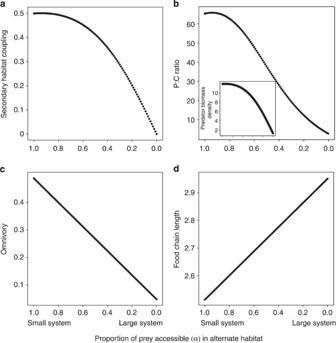Figure 2: Theoretical food web responses to changing conditions. As the system becomes effectively smaller, prey in the secondary habitat become more accessible. Macroscopic system properties change such that (a) habitat coupling increases, (b) generally the predator:consumer biomass ratio increases and predator biomass density increases (inset), (c) per cent omnivory increases and (d) food chain length decreases (for metric calculations seeMethods). Predictions are simulated using a simple spatially implicit food web model, equation (1). Predator accessibility (α) is increased (0–1). All other parameter values are held constant. Parameter values for displayed data are as follows:r=1.5,Kp=5.0,KA=5.0,eC,P=0.80, Figure 2: Theoretical food web responses to changing conditions. As the system becomes effectively smaller, prey in the secondary habitat become more accessible. Macroscopic system properties change such that ( a ) habitat coupling increases, ( b ) generally the predator:consumer biomass ratio increases and predator biomass density increases (inset), ( c ) per cent omnivory increases and ( d ) food chain length decreases (for metric calculations see Methods ). Predictions are simulated using a simple spatially implicit food web model, equation (1). Predator accessibility ( α ) is increased (0–1). All other parameter values are held constant. Parameter values for displayed data are as follows: r =1.5, K p =5.0, K A =5.0, e C,P =0.80, Full size image Our results are robust, as 100 replicates of the experiment, each with randomly chosen parameters, yielded the identical qualitative response 100% of the time, for example, an overall increasing or saturating predator density with resource accessibility, although 44% showed a hump shape response at higher resource accessibility. This humped shape outcome is not too surprising. Like other consumer resource models, reversals appear to occur at conditions near bifurcation points [33] and when exploitation rates are high (for example, high attack rates) [34] . More specifically in our model food web, near the loss of C A from the system, P begins to fall with higher α and C p is simultaneously released. In this case, C A production approaches zero and increasing predator consumption even further will quickly lead to the loss of C A from the system. Interestingly, the above conditions provide an indication of instability and extinction in our model web. Our theory generates four main predictions regarding the dependence of food web structure on the spatial properties of ecosystems (note: the results are robust to the inclusion of a switching response (unpublished data; see Supplementary Discussion )). We test spatial resource accessibility predictions against empirical web structure across two natural gradients: overall size and the relative size of littoral habitat. Food web changes across a gradient of ecosystem size Empirical data collected across a wide range in lake size (surface area min=1.10×10 2 ha, max=8.33×10 6 ha) exhibit patterns that are remarkably consistent with predictions generated from hypothesized accessibility. In agreement with the first prediction, lake trout are more strongly coupled to littoral habitats in smaller lakes ( Fig. 3a ). While biomass pyramid data are not currently available for lake trout food webs, published data from a broad sample of freshwater lakes demonstrate that biomass size spectra become more top heavy with decreasing lake size and suggest that biomass pyramids can even be inverted in small systems [35] . Biomass ratios calculated from these data show that top consumers (fish) are elevated compared with secondary pelagic consumers (zooplankton) ( Fig. 3b ) and marginally elevated for combined whole-system secondary consumer biomass (zooplankton+zoobenthos, R 2 =0.17, n =21, P =0.06) as lakes become smaller. Lake trout density data are available for a set of low productivity, unexploited, systems. In concurrence with prediction two, lake trout biomass densities in these lakes decrease as lakes increase in size ( Fig. 3b inset). The third prediction that omnivory is higher in smaller lakes is also supported by these empirical data ( Fig. 3c ). Finally, consistent with the fourth prediction the food web truncates as lake size decreases ( Fig. 3d ). 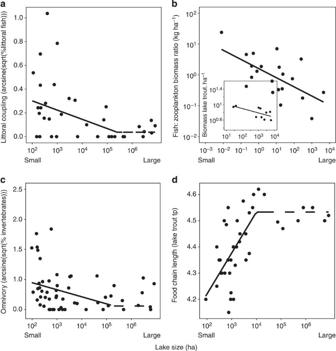Figure 3: Relationships between lake size and food webs. (a) Habitat coupling (hockey stick regression, break point=5.4,R2=0.16,n=40,P=0.036), (b) biomass ratio (linear regression,y=−0.297(log10x)+0.204,R2=0.39,n=21,P=0.002) and predator biomass density (inset) (linear regression,y=−0.11(log10x)+1.32,R2=0.42,n=10,P=0.04), (c) omnivory (hockey stick regression, break point=5.3,R2=0.12,n=56,P=0.04) and (d) food chain length (hockey stick regression, break point=4.0,R2=0.48,n=40,P=0.040). Dashed lines represent right-hand segments with slopes set to zero. Figure 3: Relationships between lake size and food webs. ( a ) Habitat coupling (hockey stick regression, break point=5.4, R 2 =0.16, n =40, P =0.036), ( b ) biomass ratio (linear regression, y =−0.297(log 10 x )+0.204, R 2 =0.39, n =21, P =0.002) and predator biomass density (inset) (linear regression, y =−0.11(log 10 x )+1.32, R 2 =0.42, n =10, P =0.04), ( c ) omnivory (hockey stick regression, break point=5.3, R 2 =0.12, n =56, P =0.04) and ( d ) food chain length (hockey stick regression, break point=4.0, R 2 =0.48, n =40, P =0.040). Dashed lines represent right-hand segments with slopes set to zero. Full size image Food web changes across a gradient of relative littoral habitat We further test our theory with a set of seven similar sized lakes from the same geographic location [30] . These lakes varied in shape such that per cent littoral habitat differs widely across lakes (% littoral area min=32, max=79). This natural experiment changes the size of the non-preferred habitat and so alters the accessibility of the near-shore zone. Furthermore, we expect that the greater the littoral area, the greater the opportunity for prey to take up refuge far from the pelagic littoral boundary and, consequently, the lower the predators' ability to consume those prey resources. Similar predictions therefore apply as lakes with small relative littoral areas should drive stronger coupling, top heavy biomass pyramids and increased omnivory. Consistent with these predictions, food webs in lakes with relatively small littoral areas are more strongly coupled ( Fig. 4a ) and exhibit more omnivory ( Fig. 4b ) than lakes with relatively large littoral areas. Food chain length and the relative littoral habitat do not vary significantly, for a linear model, but notably, in agreement with prediction four, the linear trend line slope is positive ( Fig. 4c ). For food chain length, an analysis of variance showed that a quadradic model improved fit over the linear model despite a degree of freedom penalty ( Fig. 4c ). In support of predictions, an increasing curve significantly explained the relationship ( Fig. 4c ), but with seven systems we are cautious to presume the exact shape of this relationship. 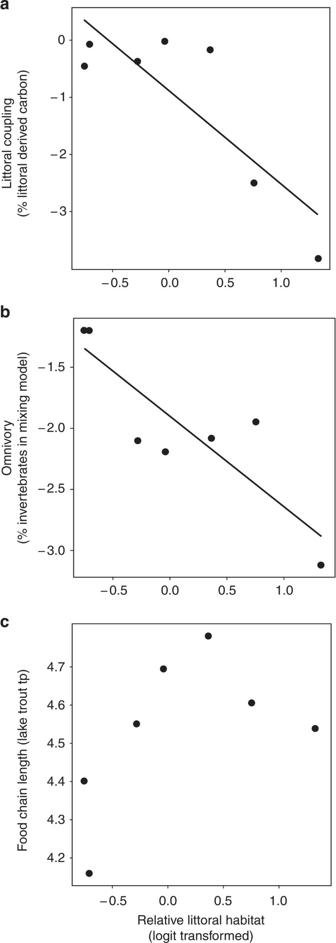Figure 4: Relationships between relative littoral habitat and food webs. (a) Habitat coupling (%) decreases (logit(y)=−1.64logit(x)−0.90,R2=0.71,n=7,P=0.03), (b) omnivory (%) decreases (logit(y)=−0.74logit(x)−1.91,R2=0.75,n=7,P=0.03), (c) food chain length increases (linear:y=0.14logit(x)+4.519,R2=0.28,n=7,P=0.2) as relative littoral habitat increases. Proportional data were logit transformed. Linear regression is used for all three statistical tests. For food chain length, an increasing quadradic model was significant (quadratic:y=0.28logit(x)−0.30(logit(x))2+4.66,R2=0.78,n= 7,P= 0.046) and was a better predictor than a straight line (analysis of variance;F=9.21, df=1,P=0.038). Structure is based on δ13C and δ15N stable isotope signatures (Methods). Figure 4: Relationships between relative littoral habitat and food webs. ( a ) Habitat coupling (%) decreases (logit(y)=−1.64logit(x)−0.90, R 2 =0.71, n =7, P =0.03), ( b ) omnivory (%) decreases (logit(y)=−0.74logit(x)−1.91, R 2 =0.75, n =7, P =0.03), ( c ) food chain length increases (linear: y =0.14logit(x)+4.519, R 2 =0.28, n =7, P =0.2) as relative littoral habitat increases. Proportional data were logit transformed. Linear regression is used for all three statistical tests. For food chain length, an increasing quadradic model was significant (quadratic: y =0.28logit(x)−0.30(logit(x)) 2 +4.66, R 2 =0.78, n = 7, P = 0.046) and was a better predictor than a straight line (analysis of variance; F =9.21, df=1, P =0.038). Structure is based on δ 13 C and δ 15 N stable isotope signatures (Methods). Full size image Little research combines theory and environmental gradients (for example, ecosystem size and temperature) to address mechanisms that influence macroscopic patterns of food web interactions and biomass structure across environmental conditions. Our theoretical food web shortened, and broadened in habitat coupling, as resource accessibility (mediated by alternate habitat size) decreased. This food web response is generally accompanied by a biomass shift from a classic Eltonian pyramid [6] to one more top heavy in shape. This general trait-mediated response is supported by empirical evidence from lake ecosystems. Further, and interestingly, omnivory and compartmentation are known stabilizing structures under the same environmental conditions in which we find them here. In large ecosystems, for example, theory shows that weak coupling to alternate compartments can allow diverse multihabitat ecosystems to persist [19] , while in small ecosystems, where interactions couple habitats so that the web behaves like a strong linear chain, omnivory is a potent stabilizing force [19] , [36] . Similarly, prey dispersal among patches in expansive systems may facilitate omnivory when top–down forces are strong enough to exclude intermediate consumers [37] . Such expansion and contraction of food web structure ought to have implications for the stability and persistence of food webs in general. These results add to an emerging literature [12] that is piecing together the role of space in food web structure and dynamics [12] , [14] , [19] , [28] , [37] , [38] . Empirical patterns show differences in food web structure across two meaningful spatial gradients that are remarkably similar to those predicted by theory. Combined, empirical data suggest that food webs are longer [20] , [22] and coupled more narrowly [30] , [39] , with lower predator biomass, in lakes where littoral resources are effectively far from the predator, and are shorter and more broadly coupled, where littoral resources are more accessible ( Fig. 4 ). Our approach differs from traditional studies in several novel ways. First, we argue that a traditional non-spatial theory would obviously not predict the same changes in omnivory, biomass structure and food chain length across systems, all else equal. Second, we limit our study to lakes with essentially the same prey trophic groups. We did this to minimize possible influences of system size on prey diversity [30] (for example, littoral coupling and omnivory in small lakes can be driven by the sheer absence of pelagic fish). Finally, coupling strength decreases with the relative littoral habitat size. As such, data support a resource accessibility theory to a greater extent than increased relative productive space, which predicts the opposite trend, or strict prey diversity arguments alone. Our findings also emphasize the notion that certain important food web structures may not be ubiquitous. Ecologists, for example, have sought compartments in food webs [24] since Gardner and Ashby [40] noted that real complex systems may persist owing to incomplete connectedness and Robert May [41] extended this result to food web compartments. Our results clearly indicate that, in nature, compartments may only exist under certain conditions. In expansive systems, we find that food chains are weakly connected across macrohabitats, and therefore are compartmentalized, whereas in small, highly connected ecosystems mobile predators strongly couple multiple energy channels and thus remove compartmentalization. Similarly, empirical studies of omnivory are somewhat conflicting [24] , [42] and are likely to be more productive if focused on assessing how omnivory, or omnivory strength, varies by following food webs in space or time. The general theory employed here argues that our results are not exclusive to lake ecosystems. On land, research from Bahamian islands suggests that smaller islands tend to have shorter food chains [7] , [26] and stronger trophic cascades [43] . From their island studies, Schoener and Spiller [43] hypothesized that refugia reduce trophic cascades on large islands. They also noticed that long points or pennisulas tend to maintain higher spider densities compared with adjacent more central habitats and suggest that these areas may be less accessed by lizard predators. It is worth mentioning that this island shape feature is analogous to long shallow bays common to lakes with large relative littoral habitat that are inaccessible to cold-water predatory fish. On the mainland, few studies link food web structure to resource conditions. A recent study shows that a balsam fir food web appears to topologically expand (that is, increase trophic position) in response to budworm outbreaks, and contract (that is, decrease trophic position) during the decline phase of the budworm cycle [44] . These collective results argue that food webs may generally expand and contract in response to changing conditions in space and time. This idea raises the question of whether modification of material pathways is fundamental for maintenance of topology, stability and thus ecosystem function in water, on land and among other ecosystem types. Furthermore, given the changing capacity of food webs, it becomes critical that we understand how human impact alters not only common food web structures but also their variability. Climate change, for example, may increase littoral temperature in northern lakes to the point that the littoral zone becomes inaccessible to cold-water fish and hence eliminates the capacity for these lake food webs to alter habitat coupling. Tools such as stable isotope analysis then take on an additional importance as a means to rapidly procure and diagnose this potential deterioration in food web structure. Isotope approaches have effectively addressed human impacts, such as the effects of flow regulation on food chain length in rivers [21] , habitat fragmentation on community niche space [45] and species invasion on food web structure [46] to name a few. Finally, we argue if food webs often change in consistent ways (for example, food chains lengthen with ecosystem size), then by identifying these consistencies, we will be in a better position to monitor food web structure and look for ecosystem-level warning signals of deleterious human change. Relationship between model and real food webs From the system outlined above, equation (1), we use functional responses to simulate (see below) measures of food web structure in the same way that empiristists use stable isotope and stomach content data to construct real webs. The theoretical model reflects a sink food web module that is commonly found in nature [16] where per cent carbon is used to delinate dependence on macrohabitats (habitat coupling), and nitrogen to determine vertical position in the web with respect to the number of trophic transfers (food chain length). In lake systems, lake trout couple a pelagic habitat channel driven by phytoplankton and a littoral habitat channel supported by attached algae and detritus [30] , [39] . Basal resources in the pelagic and littoral habitats have distinct carbon signatures making them suitable to delineate trophic groups with stable isotope approaches that also correspond to prey species habitat preferences (pelagic forage fish (for example, corigonids), pelagic invertebrates (for example, copepods), littoral forage fish (for example, cyprinids) and littoral invertebrates (for example, ephemeroptera)), and therefore make sense for use with traditional diet data as well ( Fig. 1b ; Supplementary Methods ). Thus, both our model and empirical data are posed to measure food chain length and habitat coupling width. Using the model system, we generate predator–prey interactions based on biomass flow calculated from predator functional responses. We calculate proportion of C i or R i (for example, C p P in Fig. 1c ) in predator diets simply as: Theoretical interactions where pF Px is the proportion of any single interaction (for example, F PCp ) to all interactions (∑ i F Px ) for the given web. Simulated data are comparable to empirical stable isotope or stomach contents data. As an example, a two-source isotope mixing model provides the proportion of a sample that is the sum of diet isotope signatures [47] . Stable isotope interactions where source i is the stable isotope (for example, 13 C) signature for a dietary item, and sample is predator diet [47] . We used this two-source approach to calculate habitat coupling [39] and a modified equation for food chain length [22] . For omnivory, we used a Bayesian multisource isotope mixing model (SIAR [48] ) that includes 13 C and 15 N for four dietary sources. Theoretical interactions can also be tested with traditional gut content data, although diet is not assimilated as in stable isotope analyses. Stomach content interactions Numerical simulations We performed an experiment where we simulated system dynamics over a range of spatial conditions ( α =0–1). For each condition, we sampled a time series and took the mean densities of each trophic group ( P , C 's and R 's) on the attractor between 4,000–5,000 time steps. We next determined the proportion of each prey type consumed by the top predator as a direct measure of proportional interaction strength. Four food web metrics were calculated using these simulated data: (i) habitat coupling, (ii) biomass pyramid shape, (iii) omnivory and (iv) food chain length. (i) Habitat coupling ( ω 2 ) measured here as the proportion of prey (material) consumed by the predator from the alternative habitat chain ( C A − R A ). F PCi and F PRi are the function responses for P feeding on C and R , respectively. (ii) Biomass pyramid shape ( X ) captures changes in the biomass structure among trophic levels. Here, we simply used the ratio of predators to consumer biomass density. (iii) Omnivory ( ψψ ) is determined as the resource biomass ( R 's) consumed by the predator divided by the total biomass. (iv) Food chain length ( Y ) is predicted as the trophic position of the apex predator. This method weighs the contribution of each trophic level by the relative consumption of the predator and adds 1 to account for transfer to the predator [8] . Results are shown for one parameter set (aside from manipulating α ), but are consistent over a range of parameter values. We chose the particular parameter set shown as it produced an interior equilibrium when matching parameters were set equal for both habitats. To test the generality of our findings, we ran the experiment with randomly chosen parameters until we obtained 100 parameter sets that produced an interior equilibrium ( ∼ 2,000 random sets; r i =0.01–3.0, a CiRi =0.8–2.0, a PCi =0.8–2.0, a PRi =0.0005–0.20, e =0.5–0.9, M =0.05–0.5, M Ci =0.05–0.5, K i =4.0–10.0). Essentially, this process provided 100 replicates of our experiment without species extinctions where each parameter value was selected at random. We then determined the proportion of replicates that match our predictions. Empirical analysis Our empirical analyses combined new data from recent lake surveys with data published in several studies. The ecosystem size analyses used published data [49] and added new data from a subset of lakes to calculate habitat coupling and omnivory. We only used lakes that contained a secondary consumer fish species in both habitats (pelagic fish are absent in some small lakes), so that the empirical food webs topologically match the food web model. For our new data, fish remains found in stomach contents were often not identified to species, which was used to determine habitat origin. We only added new food webs to the habitat coupling dataset when three or more species were identified for a population. Identification was not an issue for omnivory calculations, as the more coarse categories of fish or invertebrate were resolved for nearly all stomach contents. Both habitat coupling and omnivory metrics were reported as the biomass proportions of each trophic group in lake trout diets [49] ( Supplementary Methods ). We then calculated habitat coupling as the proportion of littoral fish biomass to total fish biomass (littoral + pelagic) and omnivory was calculated as the invertebrate biomass to total organisms (invertebrates + fish) in gut contents. Measures of food chain length reflect the pathways leading to a single predator (that is, a sink food web), calculated as mean lake trout trophic position, and were obtained from the literature [19] . To be consistent with recent literature that defines food chain length as maximum trophic position, recognize that lake trout often, but not always, hold the maximum trophic position in lakes. Lake trout mean trophic position is then a reasonable estimate of system food chain length for our study. This is also more likely as we excluded smaller lakes without pelagic forage where smallmouth bass ( Micropterus dolomieu ) tend to hold higher trophic positions than lake trout. We examined trophic control with biomass pyramid shape calculated using predator: consumer ratios with data from a published study [35] . To calculate this ratio, the biomass of the published trophic groups, fish, zooplankton and phytoplankton, were used. Lake trout biomass density data were collected by the Ontario Ministry of Natural Resources (OMNR) and Ministere des Resources Natural et de la Faune Quebec from calibrated netting surveys and mark recapture studies. Biomass density was calculated based on the biomass (kg) of lake trout per area (ha) of habitat. Our littoral size data are from a published study [30] and we recalculated coupling, omnivory and food chain length, again calculated as mean lake trout trophic position, according to published methods [47] . Lake characteristic details, including description of fish communities and isotope collection methods, are available from a published study [30] . For each lake, littoral habitat area proportion was calculated as the area of substrate above the 10 °C isotherm in the lake divided by the total area. Measures of δ 13 C and δ 15 N were obtained from muscle tissue samples from fish and invertebrates. Habitat coupling was calculated using a simple two-source mixing model to determine the contribution of littoral carbon to predator populations according to a previously published equation [39] ; where mean δ 13 C for predators, pelagic and littoral baseline are indicated by subscripts P , PB and LB . We used δ 13 C from Unionid mussels for the pelagic baseline and the mean δ 13 C snails and inverts as a baseline for benthic production in the littoral zone. Food chain length was calculated using mean lake trout δ 15 N and mean pelagic δ 15 N and littoral baselines δ 15 N as in coupling calculation given above [22] . To calculate omnivory, we used a Bayesian multisource mixing model, SIAR [48] , for R [50] , to determine the proportion of four dietary source groups in predator diets: zooplankton, pelagic forage fish, littoral macro invertebrates and littoral forage fish. Mean lake trout isotope values, the mean isotope values and s.d. of four dietary sources were used. Isotope values were corrected for lipid content [51] and δ 13 C (0.4±0.1) and δ 15 N (3.4±0.1) fractionation from prey to predator [47] . From these mixtures, ominvory was determined according to the theoretical metrics above, equation (8). Trends were robust over several fractionation values published for temperate lakes and lake trout systems [52] . Statistical analysis We used linear, hockey stick and quadratic regression statistical models. For the relationship between food chain length and littoral habitat proportion ( Fig. 4c ), we report quadratic regression results in addition to linear regression results and use analysis of variance to compare the two statistical models. We transformed data according to statistical requirements. Logit transforms were used for isotope proportions and littoral habitat proportions. Owing to several zero observations in the dataset, stomach content data were transformed by taking the arcsine of the square root of prey biomass proportions. How to cite this article: Tunney, T.D. et al . Food web expansion and contraction in response to changing environmental conditions. Nat. Commun. 3:1105 doi: 10.1038/ncomms2098 (2012).